Propagation stability of self-reconstructing Bessel beams enables contrast-enhanced imaging in thick media Laser beams that can self-reconstruct their initial beam profile even in the presence of massive phase perturbations are able to propagate deeper into inhomogeneous media. This ability has crucial advantages for light sheet-based microscopy in thick media, such as cell clusters, embryos, skin or brain tissue or plants, as well as scattering synthetic materials. A ring system around the central intensity maximum of a Bessel beam enables its self-reconstruction, but at the same time illuminates out-of-focus regions and deteriorates image contrast. Here we present a detection method that minimizes the negative effect of the ring system. The beam's propagation stability along one straight line enables the use of a confocal line principle, resulting in a significant increase in image contrast. The axial resolution could be improved by nearly 100% relative to the standard light-sheet techniques using scanned Gaussian beams, while demonstrating self-reconstruction also for high propagation depths. Propagation of light through inhomogeneous, disordered materials is still an enigmatic problem with unpredictable output, as complex multi-particle light scattering results in uncountable phase delays from scattered or absorbed photons. In coherent optics, strong intensity modulations arise from the interference of ballistic and diffusive photons and generate deterministic chaotic intensity distributions after some dozens of microns of propagation through scattering materials such as biological tissue. This circumstance is detrimental to image quality in light sheet-based microscopy (LSBM), where a thin plane within the sample is illuminated by a sheet of light. In the ideal but unrealistic case, the light sheet consists of purely ballistic photons, which do not interact with the various scatterers inside the sample to be imaged. However, only recently it has been shown [1] , [2] that the relative number of ballistic photons could be increased by holographically shaping the phase of the incident laser beam. This effect leads not only to enhanced penetration depths, but consequently also reduces diffusive photons or beam deflections by scattering objects. In LSBM, the light sheet is usually launched by separate illumination optics, which are oriented perpendicularly to the detection optical system, and therefore allow one to observe the propagation of illumination light through the sample. LSBM has been successfully used especially in modern developmental biology [3] or in neurology [4] , [5] . LSBM exhibits large advantages in the observation of highly dynamic (living) samples [6] , [7] , [8] , [9] , as objects are scanned plane-wise or line-wise (DSLM, digital scanned light sheet microscopy) but not point-wise as in confocal microscopy. LSBM illuminates only the part of the object that is in the plane of focus of the detection objective. As only light emerging from the focal plane is used in most imaging methods, LSBM therefore makes more efficient use of the illumination light than confocal microscopy [10] , which illuminates the whole sample for each plane that is imaged. When the illumination light propagates through a medium with an inhomogeneous refractive index distribution, scattering leads to a redistribution of light momentum and energy in the imaged plane, which causes prominent dark and bright stripes. Hence, both the light sheet quality and the image quality are deteriorated. Furthermore, spreading of the beam along the propagation direction leads to augmented illumination of out-of-focus objects thereby decreasing axial resolution and contrast for higher penetration depths. Approaches to remove background blur and to increase image contrast include structured illumination [8] , [11] , [12] and variations thereof [13] , [14] . These methods are based primarily on a removal of out-of-focus light in a post-processing step. As they require several full-frame images for each final image the acquisition speed is reduced. Furthermore, larger samples can be illuminated more homogeneously by impinging light from opposite sides [4] , [15] and scattering artefacts like stripes can be reduced by fast pivoting of the light sheet in the image plane [15] . However, all these approaches to increase image quality do not reduce light scattering and beam spreading. Although illumination by scanned Bessel beams as employed in microscopy with scanned self-reconstructing beams (MISERB) is advantageous for imaging with respect to penetration depth and directional propagation stability [16] , the accompanying ring system around their central lobe illuminates out-of-focus regions and strongly decreases contrast. In a recent study [8] it was shown that the negative effect of the rings can be avoided by using structured illumination, and/or two-photon fluorescence excitation by pulsed lasers. However, fluorescence suppression of the ring system and beam self-reconstruction in thick samples was not shown. In this paper, we show how one can block the photons emitted from the Bessel beam's ring system even in large scattering media. To remove background light from the Bessel beam's rings, we record the image line-wise so that the final image contains only that part of the object illuminated by the Bessel beam's bright central lobe. By using a confocal line detection principle, we exploit the propagation stability of the Bessel beam along one straight line (see Fig. 1 ). This approach results in a multiplication of the illumination and detection probability functions in the axial direction and therewith in a significant loss of background photons. We present a theory predicting the gain in axial resolution and show experimental results, which prove the resolution gain relative to the state-of-the-art technique using Gaussian beams. 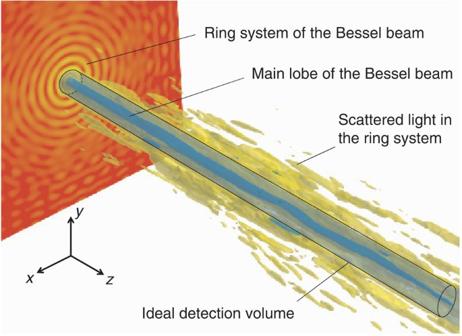Figure 1: Propagation stability of a Bessel beam. The figure shows a 3D surface plot of the intensity distribution of a Bessel beam propagating through a cluster of spheres. The data were generated by a computer simulation using the beam propagation method. The beam cross-section on the left shows the initial intensity with main lobe and ring system. The intensity of the main lobe (in blue) hardly deviates from a straight line along the propagation inzdirection due to beam self-healing. Scattering is clearly visible in the ring system (yellow). Although the ring system (in yellow) contributes background, the cylindrical outline (black) indicates the optimum volume for detecting signal-generating fluorescence photons. Figure 1: Propagation stability of a Bessel beam. The figure shows a 3D surface plot of the intensity distribution of a Bessel beam propagating through a cluster of spheres. The data were generated by a computer simulation using the beam propagation method. The beam cross-section on the left shows the initial intensity with main lobe and ring system. The intensity of the main lobe (in blue) hardly deviates from a straight line along the propagation in z direction due to beam self-healing. Scattering is clearly visible in the ring system (yellow). Although the ring system (in yellow) contributes background, the cylindrical outline (black) indicates the optimum volume for detecting signal-generating fluorescence photons. Full size image Theory We start with a closer look at the image formation process in order to understand the afore-mentioned gain in image contrast. A single beam (SB) with intensity h SB ( r ) propagating in z direction at lateral position b x =( b x ,0,0) illuminates a part of the object with three-dimensional (3D) fluorophore distribution C ( r ). The object can be displaced vertically by b y =(0, b y ,0). The resulting 3D image p SB ( r ) illuminated by a single static beam then reads The convolution (symbol) with the detection point-spread function (PSF) h det ( r ) describes the incoherent imaging process. For the conventional microscopy mode (DSLM/MISERB), the illumination beam is scanned laterally during the integration time of the sensor, h scan ( r )=∫ h SB ( r − b x ) db x producing a light sheet. The 3D image of one sheet reads If the illumination intensity h SB ( r ) corresponds to a Bessel beam, the resulting light sheet intensity h scan ( r ) is broadened considerably due to the contributions of the rings of the Bessel beam (see h scan ( y,z ) in Fig. 2a ). 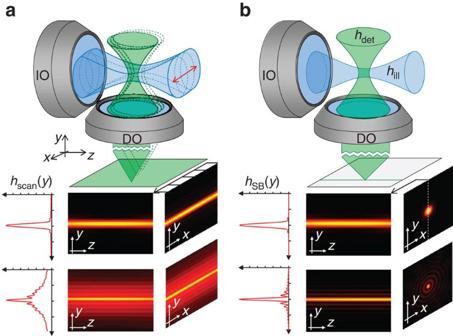Figure 2: Schematic illustration of the illumination modes. (a) Conventional light-sheet microscopy with scanned illumination beams: a beam focused by the illumination objective (IO) lens is scanned in the focal plane of the detection objective (DO) lens and a 2D image is obtained by a 2D sensor. Slices through the illumination intensity distributionhscan(y,z) andhscan(x,y) and axial profileshscan(y) are shown below for Gaussian beams (top) and Bessel beams (bottom). (b) Confocal line detection light-sheet microscope: a single-pixel line records a 1D image at the position of a single static illumination beam. The illumination intensitieshSB(y,z) andhSB(x,y) and axial profileshscan(y) are shown below for Bessel beams (top) and Gaussian beams (bottom). The non-monotonous radial decay of the Bessel beam's radial intensity profile means that the scanning substantially increases the effective thickness of the light sheet making it much thicker than the beam's central peak, as can be seen by comparing h scan ( y ) to h SB ( y ) for the Bessel beam in Figure 2 . In other words, objects below and above the focal plane of the detection objective are illuminated by a thicker light sheet, which leads to loss in image contrast. Figure 2: Schematic illustration of the illumination modes. ( a ) Conventional light-sheet microscopy with scanned illumination beams: a beam focused by the illumination objective (IO) lens is scanned in the focal plane of the detection objective (DO) lens and a 2D image is obtained by a 2D sensor. Slices through the illumination intensity distribution h scan ( y , z ) and h scan ( x , y ) and axial profiles h scan ( y ) are shown below for Gaussian beams (top) and Bessel beams (bottom). ( b ) Confocal line detection light-sheet microscope: a single-pixel line records a 1D image at the position of a single static illumination beam. The illumination intensities h SB ( y , z ) and h SB ( x , y ) and axial profiles h scan ( y ) are shown below for Bessel beams (top) and Gaussian beams (bottom). Full size image The resulting two-dimensional (2D) image obtained by an image sensor (CCD) located at y=y 0 is given by However, image contrast can be strongly increased by a confocal line principle, where only lines δ ( x−x 0 )· δ ( y−y 0 ) from 3D images p SB ( r ) at the positions of single illumination beams are collected and subsequently reassembled to a 3D image. If the central line of p SB ( r ) is selected by a line-sensor at the axial position y 0 and the lateral position x 0 , the confocal single beam (CSB) line intensity reads p CSB ( b x , b y , x 0 , y 0 , z )= p CSB ( b x , b y , z )| x 0, y 0 =∫∫ p SB ( b x , b y , x , y , z )· δ ( x−x 0 ) δ ( y−y 0 )d x d y . For a sensor in plane y 0 =0 and a line image shifted laterally by x 0 =− M · b x (with image magnification M =1 for simplicity), the image is . Insertion of p SB from equation (1) yields p CSB ( b x ,b y ,z )| bx ,0 =∫∫[∫∫∫ C ( r′ − b y )· h SB ( r′ − b x )· h det ( r − r′ )d 3 r ′]· δ ( x+b x ) δ ( y −0) d x d y . The δ -functions only affect h det and the integral reduces to It is important to emphasize that in the propagation direction z , equation (4) represents a conventional image ( C · h ill )* h det, , and a confocal image C *( h SB · h det ) in x and y directions, where the product of both the illumination PSF and the detection PSF greatly suppresses background fluorescence. A localized fluorescent probe such as a small fluorescing sphere at position r i , which is described by C ( r )= C 0 ·δ( r − r i ) allows the measurement of the effective PSF of the system. Insertion of C ( r )= C 0 · δ ( x−b x , y−b y , z ) into equation (4) delivers PSF CSB ( r ) for confocal line microscopy, while insertion into equation (3) delivers PSF LS ( r ) for a conventional light sheet system with scanned illumination beams (DSLM/MISERB): These products describe the overlap between the illumination and detection PSF. Although both products contain the same h det , the difference in the illumination, described by h SB ( x , y ,0) and h scan (0, y ,0), has a strong effect on image quality, especially for the Bessel beam that has a non-monotonously decaying radial intensity profile (see Fig. 2 ). Imaging bead clusters A flexible and well-defined way to investigate a strongly scattering sample is to use a cluster of glass or latex spheres of variable size, which can be composed in variable concentrations c . To study the propagation behaviour and suitability for imaging of Gaussian and Bessel beams, we performed measurements with fluorescent polystyrene spheres with a diameter of d= 0.75 μm (Fluoresbrite YG, Polysciences) fixed in an agarose gel cylinder at a high concentration ( c= 8×10 9 per ml). These spheres are strong scatterers due to their high refractive index of n =1.6 and sufficiently small to allow measurements of PSF LS and PSF CSB . In the following, we compare images obtained for sample illumination by scanned Gaussian beams (DSLM) and Bessel beams (MISERB) and for both beams using confocal line detection (CL-DSLM, CL-MISERB). The investigated volume of the image stacks p ( x , y , z ) was Δ x ×Δ y ×Δ z =40×10×220 μm 3 . 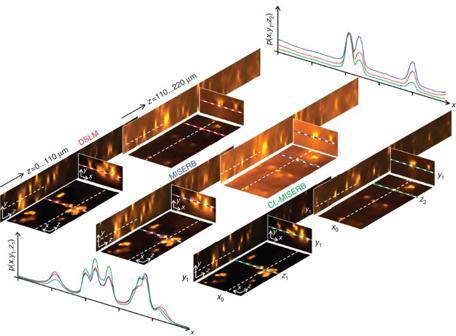Figure 3: Image slices from a cluster of fluorescent spheres. Images resulting from illumination with a scanned Gaussian beam (DSLM), a Bessel beam (MISERB) and confocal line detection for Bessel beam illumination (CL-MISERB). All white dashed lines indicate the positions where the shown image slices intersect, the coordinate is marked for the images of CL-MISERB. Vertical slicesp(x1,y,z) in the plane spanned by the illuminationzaxis and detection opticalyaxis are shown standing upright. The slices are split into two parts: one for the rangez=0–110 μm and one forz=110–220 μm. The white dashed lines (y1=6 μm) indicate the intersections with slicesp(x,y1,z) corresponding to the regular image plane. These are images from sections withz=0–35 μm andz=110–145 μm. Image slicesp(x,z1,y) andp(x,z2,y) are shown standing behind the corresponding slices. In addition, profilesp(x,y1,z) forz=z1=18.4 μm andz=z2=136.2 μm are shown for positions that are indicated by coloured dashed lines in the corresponding images with colours as follows red, blue and green represent DSLM, MISERB and CL-MISERB, respectively.. The resulting image slices p ( x,z ) (lying) and p ( y,z ), p ( x,y ) (standing) are arranged in Figure 3 . The illumination beams propagate along the z direction. The beam displacement was δx =0.4 μm, δy =0.5 μm. In general, we recorded an image p SB ( b x , x , z ) for each single static illumination beam displaced by b x , such that every image plane is composed of N= Δ x / δx= 100 images p SB ( b x , x , z ). More precisely, images in the scan mode (DSLM and MISERB) were obtained by summation over all images p SB of one plane at b y for Gaussian (DSLM) and Bessel (MISERB) beam illumination, respectively. Images p CSB ( z ) in the confocal line mode were obtained by first applying a confocal line mask with Gaussian shape to each image p SB ( b x , x, z ) and then composing all line images to a 2D image p CSB ( x , z ). The image acquisition and the calibration of the position of the confocal line mask are explained in the Methods section. In Figure 3 , white dashed lines indicate the intersections of the orthogonal image slices. In addition, coloured dashed lines indicate the positions of the intensity profiles plotted at the bottom and on top. Images p ( x , y 0 , z ) in the xy plane are shown for the image plane at y 0 =6 μm. Image slices p ( x , z ), p ( y , z ) and p ( x , y ) are shown for both a low penetration depth of the illumination beam z= (0–35) μm and for a larger penetration depth z =(110–145) μm. We extracted slices p ( x , y ) at z positions z 1 =18.4 μm and z 2 =136.2 μm. Figure 3: Image slices from a cluster of fluorescent spheres. Images resulting from illumination with a scanned Gaussian beam (DSLM), a Bessel beam (MISERB) and confocal line detection for Bessel beam illumination (CL-MISERB). All white dashed lines indicate the positions where the shown image slices intersect, the coordinate is marked for the images of CL-MISERB. Vertical slices p ( x 1 , y , z ) in the plane spanned by the illumination z axis and detection optical y axis are shown standing upright. The slices are split into two parts: one for the range z =0–110 μm and one for z =110–220 μm. The white dashed lines ( y 1 =6 μm) indicate the intersections with slices p ( x,y 1 ,z ) corresponding to the regular image plane. These are images from sections with z =0–35 μm and z =110–145 μm. Image slices p ( x , z 1 , y ) and p ( x , z 2 , y ) are shown standing behind the corresponding slices. In addition, profiles p ( x , y 1 , z ) for z = z 1 =18.4 μm and z = z 2 =136.2 μm are shown for positions that are indicated by coloured dashed lines in the corresponding images with colours as follows red, blue and green represent DSLM, MISERB and CL-MISERB, respectively.. Full size image It can clearly be seen that background is reduced by confocal line detection. The contrast improvement for CL-MISERB relative to DLSM and MISERB is especially striking in the case of higher penetration depths. The intensity profiles p ( x ) reveal the highest peaks for CL-MISERB both for z 1 =18.4 μm and z 2 =136.2 μm, whereas out-of-focus signals are blocked by CL-MISERB as in the case of the two peaks on the left side in the profile p (x, z 2 ). 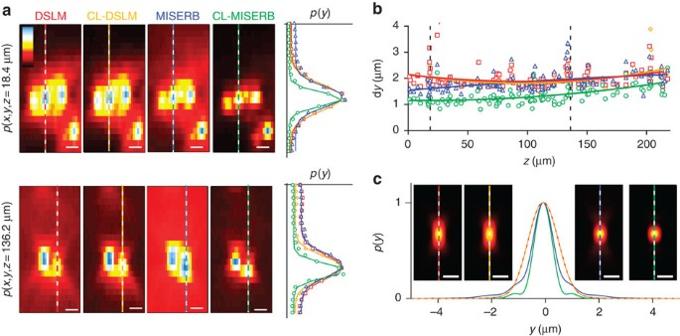Figure 4: Image slices through single spheres revealing the axial resolution. (a) For all imaging modes, slicesp(x,y) for low penetration depth of the illumination beamz=z1=18.4 μm and for largez=z2=136.2 μm are shown. Scale bar, 1 μm. The dashed lines indicate the positions of the axial profilesp(y) through one fluorescent polystyrene sphere (d=0.75 μm) that are shown on the right-hand side. The Gaussian fit function from which the axial resolution is derived is included as continuous line (DSLM is shown in red, CL-DSLM in orange, MISERB in blue, CL-MISERB in green). (b) The FWHM value dy(zi) for the line-profiles through spheresi=1–119 plotted against thezcoordinateziof the sphere it was measured for. (c) Axial intensity profilesp(y) through the image of a singled=0.75 μm sphere for all four imaging modes derived from simulated data. Furthermore, for CL-MISERB the slices p (y, z ) and p ( x , y ) show a significantly reduced extent d y of the sphere's images, that is, the PSF along the detection y axis, which is further analysed in Figure 4 . The data shown in Figure 3 illustrates that by applying the confocal line principle to each SB image p SB ( x,z ) illuminated by the Bessel beam, we could block the background photons from the Bessel ring system and thereby substantially increase image contrast. Confocal line detection also reduces the background for Gaussian beam illumination. However, images obtained by CL-DSLM and CL-MISERB reveal differences in axial resolution and signal-to-background. This is demonstrated by Figures 4 and 5 and is explained in the following. Figure 4: Image slices through single spheres revealing the axial resolution. ( a ) For all imaging modes, slices p ( x , y ) for low penetration depth of the illumination beam z = z 1 =18.4 μm and for large z = z 2 =136.2 μm are shown. Scale bar, 1 μm. The dashed lines indicate the positions of the axial profiles p ( y ) through one fluorescent polystyrene sphere ( d =0.75 μm) that are shown on the right-hand side. The Gaussian fit function from which the axial resolution is derived is included as continuous line (DSLM is shown in red, CL-DSLM in orange, MISERB in blue, CL-MISERB in green). ( b ) The FWHM value d y ( z i ) for the line-profiles through spheres i =1–119 plotted against the z coordinate z i of the sphere it was measured for. ( c ) Axial intensity profiles p ( y ) through the image of a single d =0.75 μm sphere for all four imaging modes derived from simulated data. 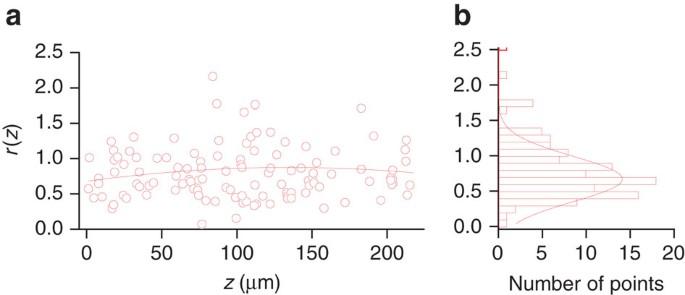Figure 5: Comparison of signal-to-background ratios. (a) Distance-dependent quotientr(z)=RDSLM/RCL−MISERBof signal-to-background ratiosR(z)=pS(z)/pBG(z) for DSLM relative to CL-MISERB and a parabolic fit. (b) Histogram of all quotientsr(z) together with a fit Gaussian function. Full size image Figure 5: Comparison of signal-to-background ratios. ( a ) Distance-dependent quotient r ( z )= R DSLM / R CL−MISERB of signal-to-background ratios R ( z )= p S ( z )/ p BG ( z ) for DSLM relative to CL-MISERB and a parabolic fit. ( b ) Histogram of all quotients r ( z ) together with a fit Gaussian function. Full size image PSF and axial resolution In incoherent imaging, the full-width at half-maximum (FWHM) of the PSF is a direct measure for the minimum resolvable distance between two adjacent points. The strong increase in axial resolution and at the same time the reduction in background by confocal line detection is illustrated in Figure 4a by images p ( x , y ) of single beads. A decrease in the axial extent of the PSF CSB ( x,y ) relative to PSF LS ( x,y )—as predicted by equations (5) and (6)—is achieved only for illumination by Bessel beams. PSF CSB and PSF LS correspond approximately to the images of the small fluorescent spheres. The line profiles p ( y )≈PSF( y ) plotted to the right of the images p ( x , y ) confirm the improvement in resolution and contrast. To obtain representative results, we analysed the images of n =119 spheres along the beam propagation distance z =0–220 μm by a software-automated extraction of the focal widths d y from the 119 axial line profiles p ( y ) for each of the four different imaging types. The centre positions ( x c , z c ) were identified manually for solitary spheres. A Gaussian function was fitted to p ( x c , i , y , z c , i ) for i= 1– n . From this fit, two parameters were extracted: first, the focal width (FWHM) as a measure for the axial resolution; second, R=p S / p BG as a measure for the signal-to-background ratio. The focal widths d y are plotted against the beam propagation distance z in Figure 4b , where least-squares parabolic fits are included for better comparability. Whereas the resolution d y is similar for scanned Gaussian (DSLM) and scanned Bessel beams (MISERB), confocal-line detection offers a substantial improvement by a factor of 1.7 for small distances z and a factor of 1.3 for large z for confocal-line detection in combination with illumination by Bessel beams (CL-MISERB). Effectively, a large part of the photons from the Bessel beam ring system is not transferred to the line detector, or, mathematically speaking, the outer parts of the intensity distribution h SB ( y ) are suppressed by the detection PSF h det ( y ), such that PSF CSB ( y )=h SB ( y )·h det ( y ) (see equation (6) becomes much narrower for the Bessel beam. The Gaussian beam, which has no rings and a broader main lobe with h SB ( y )≈ h det ( y ), is hardly affected by the removal of intensity from outer regions. It is also remarkable that no improvement is visible for confocal line detection of Gaussian beams (CL-DSLM, orange slope in Fig. 5 ) relative to DSLM (red slope). Both widths are smallest at z =110 μm, where the illumination beam h SB ( y ) is narrowest because of soft focusing with numerical aperture (NA ill )=0.07 resulting in d y =0.5 λ/NA ill =3.5 μm of the Gaussian beam. Bessel beams exhibit a stable transverse extent of the main peak along their propagation invariant depth-of-field in homogeneous space. Therefore, the focal widths of the bead images increase only slightly with z because of scattering and broadening of the thin central lobe. The broadening effect of the Gaussian beam due to scattering is less visible, as local beam distortions due to scattering are mostly within the beam's natural width, which is always larger than 3.5 μm. Nevertheless, energy is continuously taken out of the beam and results in a reduction of the peak amplitude of p ( y ), but hardly in the peak width. Signal-to-background ratio We also analysed the signal-to-background ratio R , which decreases for broader bead images p ( y ). Here, we only compared R for DSLM relative to CL-MISERB, the two other imaging modes were excluded, as they can be considered to be of minor relevance. The quotient r ( z )= R DSLM ( z )/ R CL−MISERB ( z ) is shown in Figure 5 . For a large majority of the imaged spheres, the signal-to-background is better for CL-MISERB, as indicated by r ( z )<1. The quotient r ( z ) varies strongly even for spheres at small propagation distances z . This may be explained by the different scattering behaviour of Gaussian and Bessel beams. A histogram of the n= 119 ratios r is shown in Figure 5 , revealing a mean quotient r 0 =0.64. On average, the signal-to-background ratio of CL-MISERB is factor 1/ r 0 =1.5 better than for DLSM. In summary, the results shown in Figures 2 , 3 , 4 , 5 demonstrate enhancement in image quality by confocal line detection also in the presence of beam perturbation by a scattering sample. Although image contrast is enhanced in CL-DSLM and CL-MISERB above the level of standard light sheet microscopy (DSLM), axial resolution is increased only for CL-MISERB because confocal line detection generates the signal mainly from the spatially confined central lobe of the Bessel beam. Imaging biological samples Although well-defined samples such as beads allow a reliable verification of the assumptions and comparison to theoretical calculations, 3D imaging of large biological specimens represents the main challenge to a microscope system. Therefore, we investigated fluorescence-labelled fruit fly ( Drosophila Melanogaster ) ovaries. The stage 10 egg chambers were stained with a primary antibody against the Broad protein (mouse anti-BR core 1:100, DSHB) followed by Alexa Fluor 488-conjugated secondary antibody (1:500, Molecular Probes; Fig. 6 ). In this example, two drosophila egg chambers are located behind each other (relative to the illumination direction). 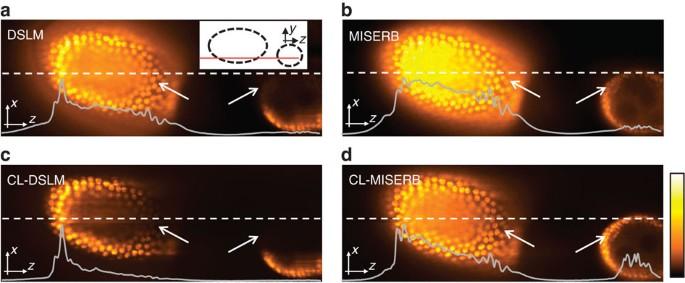Figure 6: Beam propagation and imaging of biological samples by different modes. Fluorescence images ofDrosophilaegg chambers for illumination by Gaussian beams (a,c) and Bessel beams (b,d). Illumination beams propagate from left to right. Images for scanned illumination beams are shown ina,b. Images for confocal line detection are shown inc,d. The white inset inaillustrates the vertical position of the two egg chambers and the focal plane, indicated by a red line. The grey overlays show the image intensityp(x1,z) at thexpositions marked by the dashed white lines. The size of the images shown is Δx×Δz=80×220 μm2. Both chambers are slightly displaced to each other, as indicated by the schematic inset in Figure 6a , where the red line indicates the focal plane. During image acquisition, the lateral beam sampling was δx =0.5 μm and the virtual confocal line mask width was 2 w=δx . As expected, MISERB illuminates a large number of cells inside the egg chamber located below and above the focal plane and thus delivers modest contrast ( Fig. 6b ), whereas CL-MISERB offers very good contrast all over the first (left) egg chamber ( Fig. 6d ). This is well documented by the inset intensity line profiles, which reveal a higher signal-to-background ratio as well as more details, especially—but not only—at high penetration depths. For illumination by a scanned Gaussian beam (DSLM), scattering by the first egg chamber leads to deviation and beam spreading such that the second egg chamber in the right part of the image is hardly illuminated and almost invisible (see arrow). CL-MISERB increases contrast especially at the positions marked by the arrows. This effect cannot be simply explained by the illumination geometry of Bessel beams behind an obstruction [17] . Although scattered to a large fraction by the first egg chamber to a large fraction, the Bessel beam self-reconstructs by constructive interference without significant intensity drop-off along the predicted z lines, which are selected by the confocal-line detection principle to compose the image in Figure 6d . Although CL-DSLM ( Fig. 6b ) offers the highest contrast in the left part of the object, the signal for larger penetration depth seems to be strongly reduced, with the back part of the first egg chamber becoming almost invisible (see arrow). The application of the confocal line detection principle means that hardly any light is collected in the right part of the image. The reason is the strong spreading of the Gaussian illumination beams and the bending along strong refractive index changes as, for example, the edge of the egg chamber ( Supplementary Fig. S1 ). Moreover, the Gaussian beam's spreading is so strong that the intensity illuminating the second egg chamber on the right side is too low. This result is in agreement with similar findings of Gaussian beam deflections [1] . Using the confocal line principle is therefore less useful with Gaussian beams than with Bessel beams. Figure 6: Beam propagation and imaging of biological samples by different modes. Fluorescence images of Drosophila egg chambers for illumination by Gaussian beams ( a , c ) and Bessel beams ( b , d ). Illumination beams propagate from left to right. Images for scanned illumination beams are shown in a , b . Images for confocal line detection are shown in c , d . The white inset in a illustrates the vertical position of the two egg chambers and the focal plane, indicated by a red line. The grey overlays show the image intensity p ( x 1 , z ) at the x positions marked by the dashed white lines. The size of the images shown is Δ x ×Δ z =80×220 μm 2 . Full size image Illumination efficiency Finally, we analysed the amount of light that samples are exposed to both in the experiment and simulation. Exposure of the sample to a low total light dose reduces photobleaching and phototoxic effects and is therefore crucial to live imaging over extended periods of time. To assess the light efficiency of the different microscopy methods, we evaluated the ratio η = p S / E between the usable signal amplitude p S = R p BG (see equation (6)) and the total energy delivered to the sample . An illustration can be found in Supplementary Figure S2 . E is proportional to the total fluorescence F , which can be obtained by integration of the image p ( x , y 0 , z ) in the plane y=y 0 . It was found by analysis of the data shown in Figure 3 that η DSLM / η CL-MISERB =6. This result was confirmed by a numerical analysis of the beam's intensity cross-sections ( Supplementary Fig. S3 and Supplementary Table S1 ). The result means: to obtain equal usable signal amplitudes p S in the image, the Bessel beam deposits approximately six times more energy into the sample. This is the cost for an increase in axial resolution by up to 100% ( Fig. 4 ) and in signal-to-background by 50% ( Fig. 5 ) in a sample that consists of strongly scattering beads. More details are given in the Supplementary Methods . We developed an optical method that on the one hand maintains the ring system of a Bessel beam on the illumination side, which is necessary for beam reconstruction through large and strongly scattering samples. On the other hand, the method is able to block the fluorescent photons excited by the ring system on the detection side. The confocal detection principle along a straight line offers increased contrast for both Gaussian and Bessel beams, but higher axial resolution only for Bessel beams. Furthermore, as can be seen in Figure 6 , the confocal line principle can only be applied successfully to phase shaped laser beams that hardly deflect or scatter along the propagation direction. This is the case for Bessel beams, but not for Gaussian beams. We showed that a sufficiently high number of fluorescent photons were emitted along a straight line due to excitation by ballistic photons. The composition of these 100–200 straight intensity lines per slice result in 3D image stacks with high axial resolution and contrast. The confocal line imaging principle itself requires no image post-processing, if the image is acquired line-wise. This means that resolution and contrast are enhanced already by the imaging process, as fluorescence generated by the ring system is not transferred onto the line-sensor. Furthermore, the method makes more efficient use of the dynamic range of the image sensor than structured illumination [8] , [11] or HiLo [14] , where images with modest signal-to-noise are recorded, before the signal is then improved by computational removal of the background, for example, by a linear combination of three or more modulated images. Modulation with high contrast cannot be achieved with Bessel beams because of their extended ring system, as pointed out by the intensity profile in Figure 2a . Therefore, background reduction by structured illumination for homogenous samples ( Supplementary Fig. S4 ) makes very inefficient use of the detectors dynamic range. However, the main drawback of structured illumination is that this method does not preserve high-frequency information in the image as soon as the beams forming the grid broaden due to scattering ( Supplementary Fig. S5 ), leading to dark areas in the images ( Supplementary Fig. S6 ). More details can be found in the Supplementary Methods . The increase in resolution and contrast comes at the cost of a sixfold increased sample exposure (see Supplementary Methods ). The total light dose is therefore still small in comparison to a conventional point-scanning confocal microscope that deposits over 100 times more energy into the sample to obtain a similar signal amplitude [10] . Image contrast in light sheet microscopy with Bessel beam illumination can also be increased by two-photon fluorescence excitation [8] . Because of the quadratic dependency of the fluorescence from the beam's intensity, the Bessel ring system excites a lower relative amount of fluorescence. Because of the longer wavelength used the increase in axial resolution is typically small. Moreover, it has yet to be investigated to which degree the nonlinear fluorescence excitation by Bessel beams offers an improvement in the presence of strong scattering, especially when considering pulse dispersion of the illumination light [18] , [19] . A particular strength of light sheet microscopy is the high-speed performance [7] , [8] . For the proof-of-principle measurements shown here, we used a conventional camera to record full-frame images and applied a 'line' mask in a post-processing step, which is time consuming. However, note that the total exposure time needed to achieve equal signal strength p S is the same as in the case of scanned beams (for example, MISERB) and the sum of all line images taken with the confocal line principle (for example, CL-MISERB). The image acquisition speed is solely reduced by the additional readout-time of the camera needed to transfer the full frame acquired for each beam position. By beam multiplexing, the overhead of data can be reduced and the speed increased. In combination with variable multiple region-of-interest readout by a suitable camera, significant improvements in acquisition speed could be achieved in existing setups without major changes to the hardware. A camera that allow fast 'on-the-fly' change of variable regions-of-interest would enable fast recording of line images p CSB ( z ). There are several other options to perform confocal-line detection light sheet microscopy at high speeds similar to the use of rolling-shutter cameras. Imaging at the same speed as full-frame DSLM could be enabled by integration of a line-sensor and a de-scanning mirror in the detection path. Given the options, it should soon be possible to use confocal line detection in combination with self-reconstructing illumination beams also for applications that require high image contrast at high temporal resolution. Image acquisition For proof-of-principle measurements, we implemented our confocal line method (CL-MISERB) in an existing setup without hardware changes. The microscope is equipped with long working distance water immersion objective lenses (W Achroplan ×63/0.95 and W Achroplan ×40/0.8, Carl Zeiss). The ×63 objective was used for imaging the beads. The FWHM dimensions of the PSF h det of d x =d z =0.5 μm laterally and d y =1.1 μm axially. For imaging the drosophila egg chamber, the ×40 objective was used. The Gaussian and Bessel illumination beams ( λ =488 nm) were shaped by a spatial light modulator (LC-R2500, Holoeye) so that they exhibit equal depths of field. Detailed information on the setup, sample preparation and holographic beam shaping is given in a previous publication [2] . A CCD-camera (Axiocam MRm, Carl Zeiss) is used to record full-frame-images for each lateral position x i = i ·d x of the illumination beam. The images p CSB ( z ) are obtained by multiplying the image for each beam position p i ( x , z ) with a smooth Gaussian mask m i ( x , z )=exp{−( x−x i ) 2 / w 2 } centred at the lateral position of the beam x i . Therefore x i must be known. It is possible to obtain x i either by a priori calibration or by the ex-post determination of x i from the image data. Details are given in the section on calibration below. The line width (2 w ) is ideally set to 2 w = λ /NA ill for both Gaussian and Bessel beams. As Bessel beams that exhibit identical depth-of-field as Gaussian Beams are created at higher NAs, the line width can be chosen to be much smaller for Bessel beams leading to more efficient background rejection. The final image is obtained by simple addition p CSB ( x , z )=Σ i p i ( x , z )· m i ( x , z ) of line images. For comparison, non-confocal images p LS ( x,z )=Σ I p i ( x , z ) result from using masks with w →∞ and correspond to those obtained by a scanned illumination beam (MISERB/DLSM)—except for a small constant offset due to electronic noise introduced by the detection sensor. This offset is known and can be subtracted to allow a comparison of signal-to-background ratios. Calibration Confocal line detection microscopy demands precise knowledge of the lateral beam position x i in the image plane ( xz plane). A set of n images p i ( x , z ) each shifted by d x , is taken ( i ≤ n ), so that the beam position is given by Here x off is the lateral offset position of the beam, which needs to be determined for calibration. The position of the beam is inferred from the z projection of the recorded image intensity. Either maximum selection or z integration can be used with both methods showing advantages and disadvantages in different situations. For homogeneous, extended objects (like Drosophila egg chambers), F z ,int is preferable. For isolated small objects (like microspheres), F z ,max is more robust, because F z ,int depends also on the number of fluorescent objects along z for a certain x position of the beam. 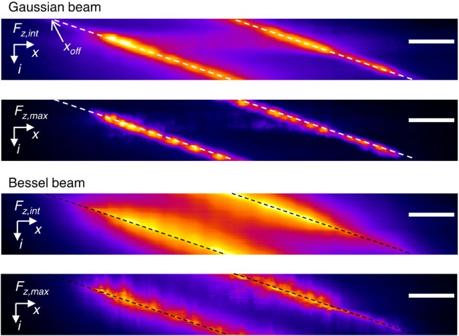Figure 7: Determination of the lateral beam positions from projections. Calibration examples forDrosophilaegg chambers are shown for Gaussian and Bessel beams. Images show the maximum intensity projectionFz,max(equation 8) and the total intensity projectionFz,int(equation 9) along the propagation axisz. The beam position index isi. The dotted lines indicate the determined beam positionxi. For confocal-line detection mode, only the small region aroundxiis used for the final image. Twofold beam multiplexing was used to increase speed. Scale bar, 10 μm. Equations (9) and (10) are illustrated by Figure 7 for image data p i ( x , z ) corresponding to the image of the Drosophila egg chamber shown in Figure 6 . The calibration consists in finding the parameters d x and x off , which are obtained by fitting a linear function to the x positions with maximum intensity extracted from F z for the n images (see dashed lines in Fig. 7 ). The procedure is substantially facilitated by the knowledge of the proportionality between the difference of the lateral beam position d x and the difference of the (voltage) signal d U applied to the scan mirror, that is, the change of the angle of the scan mirror: Figure 7: Determination of the lateral beam positions from projections. Calibration examples for Drosophila egg chambers are shown for Gaussian and Bessel beams. Images show the maximum intensity projection F z ,max (equation 8) and the total intensity projection F z ,int (equation 9) along the propagation axis z . The beam position index is i . The dotted lines indicate the determined beam position x i . For confocal-line detection mode, only the small region around x i is used for the final image. Twofold beam multiplexing was used to increase speed. Scale bar, 10 μm. Full size image Different to x off , the parameter a is very robust against drift and it is therefore sufficient to determine a only once for the setup. Thus, with d x known, the fitting procedure only needs to provide x off , which is marked by an arrow in Figure 7 . How to cite this article: Fahrbach, F.O. & Rohrbach, A. Propagation stability of self-reconstructing Bessel beams enables contrast-enhanced imaging in thick media. Nat. Commun. 3:632 doi: 10.1038/ncomms1646 (2012).